Implementation of micro-ball nanodiamond anvils for high-pressure studies above 6 Mbar Since invention of the diamond anvil cell technique in the late 1950s for studying materials at extreme conditions, the maximum static pressure generated so far at room temperature was reported to be about 400 GPa. Here we show that use of micro-semi-balls made of nanodiamond as second-stage anvils in conventional diamond anvil cells drastically extends the achievable pressure range in static compression experiments to above 600 GPa. Micro-anvils (10–50 μm in diameter) of superhard nanodiamond (with a grain size below ∼ 50 nm) were synthesized in a large volume press using a newly developed technique. In our pilot experiments on rhenium and gold we have studied the equation of state of rhenium at pressures up to 640 GPa and demonstrated the feasibility and crucial necessity of the in situ ultra high-pressure measurements for accurate determination of material properties at extreme conditions. The impact of high-pressure studies on fundamental physics and chemistry, and especially on the Earth and planetary sciences, has been enormous [1] , [2] . Compression of solids to 150–200 GPa may transform typical ionic, covalent or molecular crystals into metals and even superconductors [2] , [3] , simple metals - into optically transparent insulators [4] and change rules governing chemical processes [5] , [6] . Although experiments in diamond anvil cells (DACs) at pressures of ∼ 250–400 GPa are proven to be very difficult but possible [7] , [8] , [9] , at higher static pressures any matter has not been investigated so far. Novel shock wave techniques allow achieving pressures of hundreds of gigapascals [10] , [11] . However, at the high temperatures (thousands of degrees) and densities, generated by dynamic compression [10] , [11] , samples are in thermal equilibrium in a fluid phase. In contrast, this work deals with extending substantially the range of static pressures. Experiments conducted at static pressures have a decisive role for the investigation of phase transformations, chemical processes and the effect of compression on the structure of solids. Among various static high-pressure apparatus, only DACs provide the capability of a wide range of in situ measurements through the pressure-temperature range covering conditions over the entire Earth interior. The highest pressure, documented by X-ray diffraction studies based on the equation of state (EOS) of W reached about 420 GPa [9] by means of beveled diamonds with flat tips (culets) of about 20 μm in diameter. It seems to be not feasible achieving higher pressures without major improvement in anvils and/or design of the experiments [12] . The theory of anvils’ properties is well developed in high-pressure physics [12] , [13] . The anvils work mainly under substantial compression and must be hard, have the high compressive strength and fracture toughness. Although single-crystal diamond is anisotropic in hardness and brittle due to easy cleavage along certain crystallographic directions, it is the hardest known material with a very high compressive yield point [14] , [15] . Mechanical properties of novel nanocrystalline diamond (NCD) materials—such as, nanopolycrystalline diamond (NPD) [16] , [17] and aggregated diamond nanorods (ADNRs) [18] —are even enhanced compared with single-crystal diamonds due to suppressed anisotropy of hardness and ability for cleavage, as well as the superior fracture toughness [17] , [18] . Such excellent mechanical properties suggest that NCDs could become the material of choice for anvils, although significant luminescence of NCD limits their applications for optical studies through the anvils in DACs. It has been shown that anvils made of NPD with culets of 300–500 μm in diameter allow achieving pressures of about 1.5–2 times higher as compared with those reachable by means of single-crystal diamond anvils with the same size of the culets [19] . However, beveled anvils (the design which usually contributes to a further pressure increase), if made of NPD instead of diamond single crystals, do not show any enhancement in generation of ultra-high pressures [19] . So far a maximum pressure of 241 GPa, achieved with NPD anvils having 20 μm culets, was reported [19] . Even at moderate confining pressure of about 50 GPa the strength of diamond was documented to almost double [15] , thus potentially significantly improving the anvil’s performance. In fact, not ever proved calculations [20] suggest that the indenter-type DAC (that is, a device in which diamond with a tiny round tip is compressed against a polished diamond flat) may be able to generate pressure up to 960 GPa owing to diamond’s pressure strengthening. In order to generate pressures in the range of 0.6 TPa and above we propose to combine the advantages of NCD as anvil material and the design of a double-stage high-pressure device. In the present work we realized such a design using a conventional DAC with second-stage anvils made of NCD semi-balls. The second-stage anvils are surrounded by a pressure transmitting medium and work under significant confining pressure that allowed us to reach static pressures up to 640 GPa and accurately determine the EOS of rhenium at such extreme conditions. Synthesis and characterization of nanodiamond micro-balls We produced secondary anvils for our experiments by direct conversion of glassy carbon balls with a diameter of 20–50 μm into NCD semi-balls at 20 GPa and 2,200 K in a multi anvil press (see Methods for technical details). Depending on conditions of synthesis the balls either preserve their form ( Fig. 1 , insert) after the phase transformation into NCD (in a soft pressure medium like NaCl), or adapt more complex shapes, particularly such as semi-balls ( Fig. 2 , insert), lenses, or semi-lenses (in a hard pressure medium like MgO) with a diameter of 15 to 40 μm. X-ray diffraction, Raman spectroscopy and transmission electron microscopy (TEM) investigations confirm that the synthesized material consists of NCD with particle sizes below ∼ 50 nm (Methods, Supplementary Fig. S1 ). 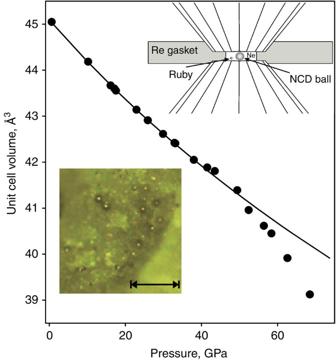Figure 1: The unit cell volume of nanocrystalline diamond (NCD) as a function of pressure. An NCD micro-ball of∼12 μm in diameter was compressed in a DAC in a Ne pressure transmitting medium (a schematic diagram is shown in insert in the upper right corner). Continues line is a result of fitting the experimental data (black dots; error bars are within the symbol size) up to 38 GPa with the third-order BM3 equation of state (K300=489(5) GPa,K′=3.2(2),V0=3.393(1) cm3mol−1). At pressures above 40 GPa the NCD seems to become more compressible, but the observed effect is simply a consequence of bridging of the micro-ball between the DAC’s anvils and the development of the deviatoric stresses in it. Insert in the bottom left shows as synthesized NCD balls (10–50 μm in diameter) in a sodium chloride medium. The scale bar is 100 μm. Figure 1: The unit cell volume of nanocrystalline diamond (NCD) as a function of pressure. An NCD micro-ball of ∼ 12 μm in diameter was compressed in a DAC in a Ne pressure transmitting medium (a schematic diagram is shown in insert in the upper right corner). Continues line is a result of fitting the experimental data (black dots; error bars are within the symbol size) up to 38 GPa with the third-order BM3 equation of state ( K 300 =489(5) GPa, K ′=3.2(2), V 0 =3.393(1) cm 3 mol −1 ). At pressures above 40 GPa the NCD seems to become more compressible, but the observed effect is simply a consequence of bridging of the micro-ball between the DAC’s anvils and the development of the deviatoric stresses in it. Insert in the bottom left shows as synthesized NCD balls (10–50 μm in diameter) in a sodium chloride medium. The scale bar is 100 μm. 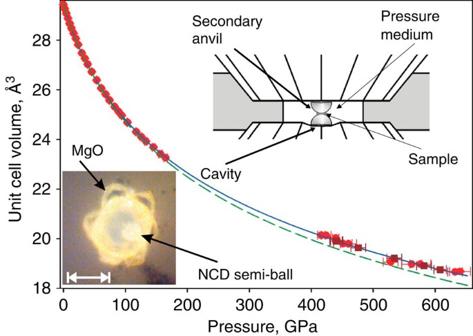Figure 2: The pressure dependence of the unit cell volume of Re. Red circles are experimental points as determined in Experiment no. 1 with the Au pressure standard26; dark-red squares are experimental points as determined in Experiment no. 2 with pressure obtained using the BM4 EOS of Re established in Experiment no. 1). Continues blue line is a result of fitting experimental data using the BM4 EOS (K300=342(6) GPa,K′=6.15(15),K″=−0.029(4), V0=29.46(1) Å3per unit cell), dashed green line is the BM3 EOS due to fitting the data collected up to 165 GPa (K300=353(3) GPa,K′=5.80(7)). Insert in the bottom left shows an example of translucent NCD semi-balls synthesized in MgO medium and used as secondary anvils, and in the upper right is a schematic drawing of the double-stage DAC assembly. The scale bar is 10 μm. A typical diameter of NCD semi-balls is 12–20 μm, and the starting size of the sample is about 3–4 μm in diameter and about 3 μm in thickness. Full size image Figure 2: The pressure dependence of the unit cell volume of Re. Red circles are experimental points as determined in Experiment no. 1 with the Au pressure standard [26] ; dark-red squares are experimental points as determined in Experiment no. 2 with pressure obtained using the BM4 EOS of Re established in Experiment no. 1). Continues blue line is a result of fitting experimental data using the BM4 EOS ( K 300 =342(6) GPa, K ′=6.15(15), K ″=−0.029(4), V 0 =29.46(1) Å 3 per unit cell), dashed green line is the BM3 EOS due to fitting the data collected up to 165 GPa ( K 300 =353(3) GPa, K ′=5.80(7)). Insert in the bottom left shows an example of translucent NCD semi-balls synthesized in MgO medium and used as secondary anvils, and in the upper right is a schematic drawing of the double-stage DAC assembly. The scale bar is 10 μm. A typical diameter of NCD semi-balls is 12–20 μm, and the starting size of the sample is about 3–4 μm in diameter and about 3 μm in thickness. Full size image First, we tested whether the NCD micro-balls really demonstrate high yield strength. In order to suppress luminescence, NCD micro-balls with a diameter of 15–20 μm were coated by a ∼ 50 nm thick gold film using a conventional sputtering technique. Then in three independent experiments they were compressed using single-crystal anvils in (100) orientation with 300-μm (in one of the experiments) or 250-μm culets ( Supplementary Fig. S2 ). To prepare a DAC, rhenium gaskets with an initial thickness of 200 μm were indented to about 30 μm, a hole with an initial diameter of 125 μm was drilled in the centre of the indentation and a gold-coated NCD micro-ball along with a small (5–8 μm in diameter) ruby ball were placed near the centre of the pressure chamber. A pressure transmitting medium (neon) was loaded into the DAC under a gas pressure of 1.2 kbar. The pressure exactly above the micro-ball ( P mb ), in proximity of the upper anvils’ culet, was evaluated from the change in the position and the shape of the high frequency edge of the diamond Raman line [21] ( Supplementary Fig. S3 ) as a result of the stress developed in the overlaying diamond anvil. The pressure around the NCD micro-ball was determined by both this method (when diamond Raman spectrum was taken above the Ne pressure medium) and by the ruby fluorescence ( P r ). As long as the NCD micro-ball does not bridge between the diamond anvils (up to about 25–40 GPa, depending on the ratio of the size of the micro-ball and the depth of the indentation in the gasket) the pressures around and exactly above the nanodiamond ball were the same. When both diamond anvils touch the NCD micro-ball, due to the gasket thickness reduction with pressure increase, the difference in the P r and P mb pressures rapidly increases in all conducted experiments and reaches the values of 48–56 GPa (before anvils or a micro-ball broke, the highest absolute value measured above the micro-ball was 97(3) GPa, whereas the pressure in the chamber determined by ruby was 41(1) GPa). The spatial resolution of the confocal Raman spectroscopy system we employed was 2 μm (see Methods) and at the highest pressure reached, the contact area between the micro-ball and the anvil was of about the same size (not larger than 4 μm in diameter). Assuming that NCD micro-balls in our experiments were under the deviatoric stress, we can estimate the maximum shear stress across the ball using the well-known relation [15] , [22] τ =1.5*( P mb − P r ). This gives 72–84 GPa as a maximum shear stress and 144–168 GPa for yield strength ( Y ) (taking in to account that Y =2* τ (ref. 14 ). These values are close to those reported [14] for the yield strength (up to 140 GPa) for the (100) diamond plane, which means that NCD micro-balls are at least as strong as single-crystal diamond. X-ray diffraction measurements on a NCD ball of ∼ 12 μm in diameter, compressed in a DAC with a Ne pressure transmitting medium using gold or neon as pressure markers [23] , reveal that up to about 38 GPa the molar volume of nanodiamond reduces monotonously ( Fig. 1 ). The experimental pressure-volume data were fitted ( Fig. 1 ) using the third-order Birch–Murnaghan (BM3) EOS: where P is pressure; V is the volume at pressure P ; K 300 , K ′, K ″ and V 0 are the bulk modulus, its first and second pressure derivatives, and the volume at zero pressure, correspondingly. This fitting procedure gave the values of K 300 =489(5) GPa, K ′=3.2(2), V 0 =3.393(1) cm 3 mol −1 , which within the uncertainty limits coincide with the data from Dubrovinskaia et al . [24] for ADNRs. At pressures above 40 GPa the NCD seems to become more compressible ( Fig. 1 ), but the observed effect is simply a consequence of bridging of the micro-ball between the DAC’s anvils and the development of the deviatoric stresses in it. As follows from Fig. 1 and the NCD EOS, at 68 GPa in the pressure chamber determined on the ruby standard, stress on the micro-ball reaches 44 GPa (indeed, if pressure would be calculated based on extrapolation of the NCD EOS (solid line in Fig. 1 ), one could judge it as equal to 112 GPa for the same NCD unit cell volume as that measured at 68 GPa). However, observed splitting of Ne diffraction lines in the patterns collected through the ball at the point of its contact with the diamond anvil ( Supplementary Fig. S4 ) may indicate that the stress distribution (or Ne behaviour under stress) is more complex and perhaps cannot be described in a simple uniaxial model. Detailed analysis of these observations is outside the scope of the current work and will be presented elsewhere. Static compression experiments above 600 GPa After establishing that the synthesized NCD has a high yield strength and is less compressible and less brittle than single-crystal diamonds, we employed the NCD semi-balls as second-stage anvils in DACs ( Fig. 2 , insert; Supplementary Fig. S5a ). Numerous trial and error experiments resulted in some empirical observations regarding the behaviour of the second-stage anvils: (a) the second-stage anvils placed at the primary anvil have the tendency to shift upon pressure increase, thus destroying the alignment. In order to avoid this problem we fixed the NCD semi-balls in a small cavity made on the surface of the diamond anvil by a pulsed laser ( Supplementary Fig. S5b ). (b) If the second-stage anvils bridge between the primary ones at pressure in the chamber below 30–35 GPa, the NCD semi-balls glide over each other. This limits the lower bound of pressure possible to be generated using the double-stage DACs at the moment. (c) If a sample has a bigger size than the contact area between the second-stage anvils, the latter also demonstrate a tendency to glide. We conducted two successful experiments with the double-stage DACs, which were prepared, loaded and compressed at BGI (Bayreuth, Germany) to that extent that the contact between the second-stage anvils was achieved. Subsequently the DACs were transferred to the 13-IDD station at the Advanced Photon Source (USA) for synchrotron X-ray powder diffraction measurements with a beam focused down to <4 μm in diameter at 0.3344 Å wavelength. Choice of the pressure standard is one of the most important issues in any high-pressure experiment. The pressure dependence of the lattice parameters (the molar volumes) of the markers is at present the only available method to characterize pressures in the 500 GPa range, because there are no optical sensors calibrated at these required pressures. Gold is probably one of the best standards for ultra-high pressures. It does not undergo phase transitions upon compression up to at least 275 GPa at ambient temperature [25] , its EOS based on diffraction data collected in DACs is the focus of continuing investigations by various research groups that resulted in consistent data sets (see Fei et al . [23] and references therein), and the EOSs from dynamic (shock wave) experiments at 0.55 TPa range [26] agree well with those based upon static data [23] . In the first of our experiments powders of rhenium and gold were mixed together and the mixture was placed between the NCD anvils of the second stage. Gold was used as a pressure standard and the EOS of rhenium was determined. The lattice parameters of gold measured in this experiment ranged from 3.4091(5)–3.303(3) Å ( Figs 2 and 3 ; Table 1 , Experiment no. 1) corresponding to the pressure range between 416(4) and 640(17) GPa according to the gold EOS [26] . Experiment no. 2 ( Table 1 ) was conducted on pure Re, because it turned that the amount of gold, which was mixed with Re and put between the second-stage anvils was insufficient for obtaining gold diffraction. For this reason we used the EOS of Re obtained in Experiment no. 1 to determine pressure in Experiment no. 2 and found that we were able to compress the sample to 608 (7) GPa ( Fig. 2 ; Table 1 , Experiment no. 2). Even at the highest pressure reached we did not see signs of significant deviatoric stresses on the sample and could accurately determine lattice parameters ( Table 1 ) using the GSAS programme. Diffraction from the second-stage anvils appeared to be very weak at ∼ 400 GPa and became effectively not detectable at higher pressures, probably fully hidden under reflections of heavy metals (samples containing Au and Re). In the experiments in the double-stage DACs we used paraffin (Experiment no. 1) and solid Ne (Experiment no. 2) as a pressure medium surrounding secondary anvils with the sample. Similarly to the experiments with NCD micro-balls described above, relatively small changes in pressure within the pressure medium (33–58 GPa) resulted in a huge pressure increase on a sample placed between the secondary anvils (up to 640 GPa) ( Supplementary Fig. S6 ). 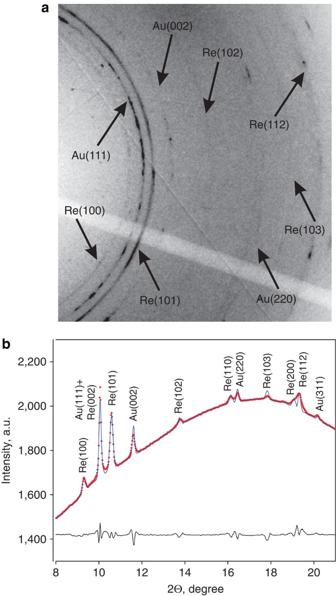Figure 3: The synchrotron powder X-ray diffraction data of a mixture of Re and Au. (a) A part of the 2D X-ray diffraction image. (b) The GSAS plot. The data were collected at an X-ray wavelength ofλ=0.3344 Å and at a pressure of 640(17) GPA. Red dots are the experimental data, the blue curve is the simulated diffraction data and the dark line is the residual difference. A mixture of Au and Re powders was compressed in a double-stage DAC using paraffin as a pressure transmitting medium. The lattice parameter of gold isa=3.303(3) Å, and those of rhenium area=2.382(1) Å andc=3.798(2) Å. Pressure was determined according to the gold equation of state26. Figure 3: The synchrotron powder X-ray diffraction data of a mixture of Re and Au. ( a ) A part of the 2D X-ray diffraction image. ( b ) The GSAS plot. The data were collected at an X-ray wavelength of λ =0.3344 Å and at a pressure of 640(17) GPA. Red dots are the experimental data, the blue curve is the simulated diffraction data and the dark line is the residual difference. A mixture of Au and Re powders was compressed in a double-stage DAC using paraffin as a pressure transmitting medium. The lattice parameter of gold is a =3.303(3) Å, and those of rhenium are a =2.382(1) Å and c =3.798(2) Å. Pressure was determined according to the gold equation of state [26] . Full size image Table 1 Pressure dependence of the unit cell parameters of hcp- Re as determined in DACs experiments. Full size table Although the behaviour of rhenium at high pressure has been investigated extensively by experimental (shock wave, X-ray powder and radial diffraction in DACs, ultrasonic measurements) and theoretical methods, there is a lack of consistency on its ambient temperature EOS [9] , [22] , [27] , [28] . Although ab initio calculations resulted in a broad range of bulk moduli (344–447 GPa, see Duffy et al . [27] and references therein), different experiments are in reasonable agreement regarding K 300 (350–372 GPa) but highly diverse in reported values of K ′ (2.93–5.43, see refs 9 , 22 , 27 , 28 ). Moreover, Jeanloz et al . [22] proposed the fourth order BM (BM4) EOS for rhenium based on combined ultrasonic data and Hugoniout measurements up to 170 GPa, but it demonstrates unphysical behaviour above 240 GPa ( Supplementary Fig. S7 ). These discrepancies may be resolved based on our measurements at pressures above 400 GPa, if they would be combined with the low pressure data set. Complementary to the ultra high-pressure experiments in double-stage DACs, we compressed Re powder in a He pressure medium in a conventional DAC (Experiment no. 3) with beveled diamonds (120 μm culets) using Au as a pressure marker ( Fig. 2 and Table 1 , Experiment no. 3). The experimental data collected between ambient conditions and 165 GPa ( Fig. 2 ) may be described by the BM3 EOS (see equation (1)) with the parameters K 300 =353 (3) GPa, K ′=5.80(7) and V 0 =8.87(1) cm 3 mol −1 (or equally well by the Vinet EOS: with the parameters K 300 =348(5) GPa, K ′=7.57(7), V 0 =8.87(1) cm 3 mol −1 ). However, extrapolation to higher pressures using both the BM3 and Vinet EOSs failed to reproduce data collected at pressures between 400 and 640 GPa. Indeed, at the highest pressure of 640 GPa, the BM3 EOS misfits the experimental data by >10% (pressure underestimate is about 70 GPa) ( Supplementary Fig. S8 ). The data-points at pressure up to 165 GPa are not sufficient to constrain the BM4 EOS, and only by combining the results obtained in conventional and double-stage DACs ( Table 1 ) we can fit the whole available data set with the unique BM4 EOS: where K 300 =342(6) GPa, K ′=6.15(15), K ″=−0.029(4), V 0 =8.87(1) cm 3 mol −1 ( Fig. 2 ; Supplementary Fig. S7 ). Thus, we not only demonstrate the necessity of using the fourth order BM4 EOS in order to describe properly the behaviour of Re at high pressure, but also establish that for such a low-compressible material as rhenium static compression data in the 0.5 TPa range are essential. Of course, numerical parameters of the EOS depend on a pressure standard used (gold in our case) and the unknown systematic uncertainty is inherent in choosing one of many available EOSs (see Table 1 ). The extension of the accessible pressure range above 500 GPa requires further development of self-consistent experimentally determined pressure standards [23] . Previous experimental and theoretical studies indicated that the c/a lattice parameters ratio of hexagonal close-packed ( hcp ) structured Re stays fairly constant up to about 200 GPa [28] , [29] , [30] , while ab initio simulations predicted complex nonlinear variations (although small, within 0.33%) in the 1 TPa pressure range [31] . Our data collected in He (Experiment no. 3), a quasi-hydrostatic pressure transmitting medium, shows that at pressures below 120 GPa the c/a is actually constant within the measurement uncertainties, but at higher pressures up to 165 GPa the c/a slightly decreases (by <0.2%). At the much higher pressures achieved in the double-stage DACs, the c/a ratio of hcp -Re decreases significantly (compare 1.615 at ambient pressure to 1.595 (1.3%) at 640 GPa, Supplementary Fig. S9 ), thus qualitatively supporting theoretical predictions [31] . In the present work we have demonstrated that double-stage DACs with secondary anvils fabricated from NCDs allow to drastically extend the achievable pressure range in static compression experiments. Feasibility of the technique was demonstrated in pilot experiments at pressures above 600 GPa. In the future, implementation of computer controlled micromanipulators for mounting of the secondary anvils and assembly of the samples, as well as preparation of the samples using the focused ion beam (FIB) or deposition techniques, would allow improving the stability of the high pressure cells for static ultra high-pressure investigations. Moreover, advantages due to optimization of the shape of the secondary anvils and choice of nanodiamonds with different crystallite sizes and shapes [16] , [24] are yet to be explored. Thus, we are confident that achieving 1 TPa in static compression experiments with double-stage DACs is a viable goal. Materials As starting material for the synthesis of NCD in shapes of balls, semi-balls and lenses we used glassy carbon balls with a diameter of 20–50 μm (Alfa Aesar GmbH). Gold powder (99.9995% purity, 1 μm particle size) and rhenium powder (99.99% purity, 5 μm particle size) were purchased from Goodfellow Inc. Fabrication of nanocrystalline balls and semi-balls Nanocrysatlline balls, semi-balls and NCD with other shapes were fabricated in a 5,000-ton multi-anvil press using glassy carbon balls as starting materials. The glassy carbon balls were mixed either with NaCl or MgO, and the samples were enclosed into a h-BN capsule. The sample assembly consisted of a MgO (+5 wt% Cr 2 O 3 ) octahedron (18 mm edge length) containing a LaCrO 3 heater. The octahedron was compressed using 54 mm tungsten carbide anvils with a truncation edge length of 11 mm and pyrophyllite gaskets. The temperature was monitored with a W 3 Re/W 25 Re thermocouple located axially with respect to the heater and with a junction close to the h-BN capsule. Experiments were conducted at pressure of 20 GPa and temperature up to 2,200 K. The P–T uncertainties are estimated to be ±1 GPa and ±50 K, respectively. In each experiment the sample was first compressed to the desired pressure; the temperature was then raised at ∼ 100 K min −1 to the desired run temperature. Duration of heating varied from several minutes to 15 min. The samples were either quenched by switching off the power to the furnace, or gradually cooled with a rate of ∼ 10 K min −1 , and then slowly decompressed. Upon completion of each experiment, the capsule was carefully removed and the treated material was mechanically cleaned to remove BN. Synthesized NCD materials were cleaned from NaCl in water and from MgO in a 1-M solution of HCl. Depending on the synthesis conditions, glassy carbon balls either preserved their form (in soft pressure medium like NaCl) or turned to more complex shapes (in hard pressure medium like MgO). DAC experiments For all our experiments we used piston-cylinder type DACs with a large optical aperture produced at BGI. Diamonds with culet sizes of 250 or 300 μm were used in conventional DAC experiments or as primary anvils. Compression of Re powder in a He pressure medium to 165 GPa was conducted with beveled diamonds with 120 μm culets. As gasket materials Re or Ir were employed. Gaskets were indented to the thickness of 20–35 μm in different experiments and holes with a diameter of 125–150 μm were drilled in the centre of the indentation. As a pressure transmitting medium He and Ne was loaded at pressure of 1.2 kbar, and in some experiments with double-stage DACs liquid paraffin was used. Cavity in diamond anvils for experiments with double-stage DACs were made by a picosecond pulsed laser. X-ray diffraction measurements We conducted in situ X-ray high-pressure experiments at the Bayerisches Geoinstitut (Germany), at ID09 ESRF (France), and at 13-IDD at Advanced Photon Source (APS), USA. At the Bayerisches Geoinstitut we obtained powder X-ray diffraction data with a system consisting of a Rigaku FRD high-brilliance generator (90 kW) and APEX CCD Area Detector. The Mo K α radiation (tube voltage 60 kV, tube current 55 mA, cathode gun 0.1 × 0.1 mm 2 ) was focused with MaxFlux X-ray optics and further collimated down to ∼ 30 μm FWHM beam size. At the ID09 at ESRF the data were collected with the MAR555 detector using the X-ray beam of ∼ 0.41 Å wavelength and a size of beam down to 5 × 5 μm 2 . All experiments with double-stage DACs were performed at 13-IDD station (GSECARS) using a MAR-165 CCD area detector and a highly focused beam ( ∼ 3 × 4 μm 2 ) of 0.3344 Å. The collected images were integrated using the Fit2D or GADDS programs in order to obtain a conventional diffraction pattern ( Supplementary Fig. S10 ). Data analysis was conducted using the GSAS package [32] , [33] . Raman spectroscopy Raman spectroscopy was used in order to measure ruby fluorescence and stress in the diamonds over compressed nanocrystalline microspheres. Measurements were performed with the LabRam and Dilor XY (DILOR GmbH) systems with a resolution better than 2 cm −1 . With a X50 long working distance objective and confocal optics employed, the spatial resolution was ∼ 2 μm. The 632.8 nm line of a He–Ne laser and 514 nm of an Ar laser were used for an excitation with a power at the sample position of 15–50 mW. The positions of the fluorescence lines and Raman peaks were determined by processing experimental data using PeakFit v4.12 software. Transmission electron microscopy A TEM specimen of a NCD semi-ball was prepared by the FIB technique on a FEI Helios NanoLab 650 instrument. Electron diffraction patterns and conical dark field images were recorded on a FEI Tecnai G2 microscope operated at 200 kV. Electron energy loss spectra (EELS) were obtained on a FEI Titan 80–300 microscope operated in scanning TEM mode at 120 kV and equipped with a GIF QUANTUM spectrometer as well as an aberration corrector fro the probe-forming lens. The convergence semi-angle α was ∼ 21 mrad, the acceptance angle β was ∼ 50 mrad. The electron diffraction patterns ring pattern of the NCD semi-ball FIB slice displays diffraction rings typical for the f.c.c. diamond structure with a≈ 3.57 Å ( Supplementary Fig. S1 ). Conical dark field TEM images, taken with the 111 diamond reflection ring, demonstrate that the NCD semi-ball consists of randomly oriented diamond nano-crystals with a rather uniform size. The crystal size varies from 3–55 nm with a mean value of 21 (10) nm. EELS spectra taken from many particles simultaneously reveal that the sample contains almost pure sp 3 -hybridized carbon ( Supplementary Fig. S11 ). Almost no π* contribution, typical of sp 2 -hybridized carbon, can be measured indicating that its content in the material is extremely low. How to cite this article: Dubrovinsky, L. et al . Implementation of micro-ball nanodiamond anvils for high-pressure studies above 6 Mbar. Nat. Commun. 3:1163 doi: 10.1038/ncomms2160 (2012).